Stargazin regulates AMPA receptor trafficking through adaptor protein complexes during long-term depression Long-term depression (LTD) underlies learning and memory in various brain regions. Although postsynaptic AMPA receptor trafficking mediates LTD, its underlying molecular mechanisms remain largely unclear. Here we show that stargazin, a transmembrane AMPA receptor regulatory protein, forms a ternary complex with adaptor proteins AP-2 and AP-3A in hippocampal neurons, depending on its phosphorylation state. Inhibiting the stargazin–AP-2 interaction disrupts NMDA-induced AMPA receptor endocytosis, and inhibiting that of stargazin–AP-3A abrogates the late endosomal/lysosomal trafficking of AMPA receptors, thereby upregulating receptor recycling to the cell surface. Similarly, stargazin’s interaction with AP-2 or AP-3A is necessary for low-frequency stimulus-evoked LTD in CA1 hippocampal neurons. Thus, stargazin has a crucial role in NMDA-dependent LTD by regulating two trafficking pathways of AMPA receptors—transport from the cell surface to early endosomes and from early endosomes to late endosomes/lysosomes—through its sequential binding to AP-2 and AP-3A. The AMPA (α-amino-3-hydroxy-5-methyl-4-isoxazole propionic acid)-type glutamate receptor mainly mediates fast excitatory neurotransmission in the vertebrate central nervous system [1] . The accumulated evidence indicates that long-lasting synaptic plasticity in the form of long-term potentiation and long-term depression (LTD) results, respectively, from the regulation of the exocytosis and endocytosis of postsynaptic AMPA receptors, which is induced by neuronal activity [2] , [3] . The trafficking of membrane proteins is generally achieved by vesicle carriers that selectively sort cargo proteins via various adaptor proteins (APs), such as the tetrameric AP complexes, AP-1, AP-2, AP-3 and AP-4 (ref. 4 ). For example, in mammalian cells the clathrin-mediated endocytosis of cell surface proteins is mainly regulated by AP-2, whereas the delivery of cargo proteins from early endosomes to late endosomes and/or lysosomes is mediated by AP-3A [5] . Although the μ2 subunit of AP-2 is reported to bind to AMPA receptor subunits GluA2 and GluA3 (refs 6 , 7 ), it has been unclear whether and how this process is regulated by neuronal activity. Furthermore, although after their endocytosis, the AMPA receptors are known to be trafficked to the late endosomal and/or lysosomal pathway [8] , [9] , [10] , whether and how this process is causally involved in LTD is not well understood. Transmembrane AMPA receptor regulatory proteins (TARPs) are tightly associated with AMPA receptor subunits and are essential for the function of synaptic AMPA receptors [11] . In addition, activity-dependent dephosphorylation of stargazin (STG), a prototypical TARP, by the NMDA ( N -methyl- D -aspartate) receptor-mediated activation of calcineurin has a crucial role for low-frequency stimulus (LFS)-induced LTD in the hippocampus [12] . Recently, the phosphorylation of STG was shown to be necessary for its dissociation from negatively charged lipid bilayers and subsequent binding to the anchoring protein PSD-95 at postsynaptic sites [13] . However, it remains unclear how STG regulates endocytosis of postsynaptic AMPA receptors during LTD. We previously showed that the μ-subunit of AP-4 binds to the carboxy terminus of STG and regulates the polarized transport of the AMPA receptor–STG complex to the somatodendritic domain of neurons [14] . As the μ-subunits of various AP complexes often recognize similar binding motifs within cargo proteins [15] , we hypothesized that postsynaptic AMPA receptor trafficking might be generally regulated by interactions between TARPs and various AP complexes. In the present study, we find that AP-2 and AP-3A bind strongly to the dephosphorylated but not phosphorylated STG. Disrupting the association between STG and AP-2 blocks NMDA-dependent AMPA receptor endocytosis and LFS-induced LTD in the hippocampus. Furthermore, when the interaction between STG and AP-3A is inhibited, the endocytosed AMPA receptors reappear on the surface of hippocampal neurons and the LFS-induced LTD is inhibited. These results indicate that during LTD, the NMDA receptor-mediated activation of calcineurin dephosphorylates STG, which first binds to AP-2 to induce the clathrin-dependent endocytosis of AMPA receptors, and then binds to AP-3 to deliver AMPA receptors to the late endosomes/lysosomes. STG recruits AP-2 and AP-3A to the AMPA receptor complex To test the hypothesis that STG binds to AP complexes besides AP-4, we first purified the C terminus of STG as a glutathione S -transferase (GST) fusion protein and performed pull-down assays using cell lysates of human embryonic kidney 293 (HEK293) cells expressing the μ-subunit of AP-2 (μ2), AP-3A (μ3A) and AP-4 (μ4). As reported for μ4 (ref. 14 ), the μ2 and μ3A subunits robustly bound to GST–STG ( Fig. 1a , left panels). The amount of μ-subunits pulled down by GST itself was similar to that observed without using any GST proteins ( Fig. 1a , right panels), indicating that these weak signals are caused by nonspecific binding of μ-proteins to glutathione sepharose beads. The middle part of the C terminus of STG, which we refer to as the CT2 region, was previously shown to be responsible for the interaction between μ4 and STG [14] . As with μ4, GST–STG lacking the CT2 region (STG ΔCT2 ) did not bind to μ2 or μ3A ( Fig. 1a , left panels). To further examine whether μ2 could directly interact with STG in a cell-free system, we purified μ2 as a fusion protein with maltose binding protein (MBP-μ2). GST pull-down assays revealed that MBP-μ2 bound to GST–STG wt , but not to the mutant GST–STG ΔCT2 ( Fig. 1b ). Furthermore, a co-immunoprecipitation assay showed that the μ2 and μ3A subunits associated with STG (γ2) and with other TARPs (γ3, γ4 and γ8) in HEK293 cells ( Supplementary Fig. S1a,b ). These results indicate that the CT2 region of STG, and possibly of other TARPs, binds to AP-2 and AP-3A. 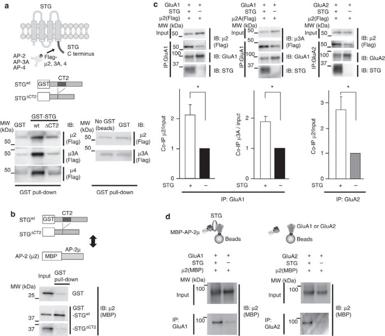Figure 1: STG mediates the formation of a ternary complex with AP-2 and AP-3. (a) The binding of STG’s C terminus to APs-2, -3 and -4 is dependent on its CT2 region. Lysates of HEK293 cells expressing Flag-tagged μ2, μ3A or μ4 subunits were pulled down by glutathione beads alone, GST, the GST-tagged C terminus of STG (GST–STGwt) or a GST–STG mutant lacking the CT2 region (GST–STGΔCT2), and immunoblotted (IB) with an anti-Flag antibody. A part ofFig. 3cis shown on the right panels to illustrate the background binding of glutathione beads and GST to μ2 or μ3A. (b) Purified μ2 binds directly to STG in a manner requiring STG’s CT2 region. μ2 was purified as a fusion protein with MBP-μ2, pulled down by GST, GST–STGwtor GST–STGΔCT2, and immunoblotted (IB) with an anti-MBP antibody. (c) Co-immunoprecipitation assays showing blotting results above and quantification in bar graphs below. For the bar graphs, the intensity of the band corresponding to μ2 or μ3A that was co-immunoprecipitated was normalized to the intensity of the respective molecule in the input lysate. The value in the absence of STG was arbitrarily established as 1.0. Coexpression of STG strongly enhanced the co-immunoprecipitation of μ2 (left panel) or μ3A (middle panel) with GluA1 and μ2 with GluA2 (right panel). Lysates of HEK293 cells expressing GluA1/GluA2 and Flag-tagged μ2/μ3A with or without STG were immunoprecipitated using an anti-GluA1 or anti-GluA2 antibody and immunoblotted with anti-Flag, anti-GluA1 or anti-GluA2 and anti-STG antibodies (n=5, experimental replicates). *P<0.05 by Student’st-test. Error bars represent means+s.e.m. (d) Purified μ2 binds to the AMPA receptor complex via STG in a cell-free system. Lysates of HEK293 cells expressing GluA1 alone or GluA1 plus STG were immunoprecipitated by an anti-GluA1 antibody and purified MBP-μ2 was added to the precipitated fraction. Immunoblot analysis using an anti-MBP antibody revealed that purified MBP-μ2 bound to the GluA1–STG complex but not to GluA1 alone (left panels). Similarly, MBP-μ2 bound to the GluA2–STG complex but not to GluA2 alone (right panels). Figure 1: STG mediates the formation of a ternary complex with AP-2 and AP-3. ( a ) The binding of STG’s C terminus to APs-2, -3 and -4 is dependent on its CT2 region. Lysates of HEK293 cells expressing Flag-tagged μ2, μ3A or μ4 subunits were pulled down by glutathione beads alone, GST, the GST-tagged C terminus of STG (GST–STG wt ) or a GST–STG mutant lacking the CT2 region (GST–STG ΔCT2 ), and immunoblotted (IB) with an anti-Flag antibody. A part of Fig. 3c is shown on the right panels to illustrate the background binding of glutathione beads and GST to μ2 or μ3A. ( b ) Purified μ2 binds directly to STG in a manner requiring STG’s CT2 region. μ2 was purified as a fusion protein with MBP-μ2, pulled down by GST, GST–STG wt or GST–STG ΔCT2 , and immunoblotted (IB) with an anti-MBP antibody. ( c ) Co-immunoprecipitation assays showing blotting results above and quantification in bar graphs below. For the bar graphs, the intensity of the band corresponding to μ2 or μ3A that was co-immunoprecipitated was normalized to the intensity of the respective molecule in the input lysate. The value in the absence of STG was arbitrarily established as 1.0. Coexpression of STG strongly enhanced the co-immunoprecipitation of μ2 (left panel) or μ3A (middle panel) with GluA1 and μ2 with GluA2 (right panel). Lysates of HEK293 cells expressing GluA1/GluA2 and Flag-tagged μ2/μ3A with or without STG were immunoprecipitated using an anti-GluA1 or anti-GluA2 antibody and immunoblotted with anti-Flag, anti-GluA1 or anti-GluA2 and anti-STG antibodies ( n =5, experimental replicates). * P <0.05 by Student’s t -test. Error bars represent means+s.e.m. ( d ) Purified μ2 binds to the AMPA receptor complex via STG in a cell-free system. Lysates of HEK293 cells expressing GluA1 alone or GluA1 plus STG were immunoprecipitated by an anti-GluA1 antibody and purified MBP-μ2 was added to the precipitated fraction. Immunoblot analysis using an anti-MBP antibody revealed that purified MBP-μ2 bound to the GluA1–STG complex but not to GluA1 alone (left panels). Similarly, MBP-μ2 bound to the GluA2–STG complex but not to GluA2 alone (right panels). Full size image Although AMPA receptors do not bind directly to AP-4, their somatodendritic trafficking is regulated by forming a tripartite complex with STG and μ4 (ref. 14 ). Therefore, we next used a co-immunoprecipitation assay to examine whether AMPA receptors and STG can also form a ternary complex with μ2 or μ3A. Flag-tagged μ2 or μ3A and GluA1 or GluA2 were coexpressed with or without STG in HEK293 cells. The amount of μ2 or μ3A that co-immunoprecipitated with GluA1 or GluA2 increased significantly when STG was coexpressed ( Fig. 1c ). When GluA1 or GluA2 was not coexpressed in HEK293 cells, only a very small amount of μ2 or μ3A proteins were co-immunoprecipitated by GluA1 or GluA2 antibodies ( Supplementary Fig. S1c ). Non-immune IgG also failed to immunoprecipitate the μ2 or μ3A protein ( Supplementary Fig. S1d ). Finally, actin protein did not co-immunoprecipitate with GluA1 in the presence or absence of STG ( Supplementary Fig. S1d ). These results suggest that STG mediates the formation of a complex between AMPA receptor and AP-2 or AP-3. It is possible that the facilitatory effect of STG on the interaction between AMPA receptor and μ2 was not caused by a direct interaction between STG and μ2, but was instead mediated by the increased surface trafficking of AMPA receptors in the presence of STG. Thus, we next examined whether purified μ2 could directly bind to GluA1 or to the GluA1–STG complex in a cell-free system. Lysates of HEK293 cells expressing GluA1 alone or GluA1 plus STG were immunoprecipitated by an anti-GluA1 antibody and purified MBP-μ2 was added to the precipitated fraction. Immunoblot analysis using an anti-MBP antibody revealed that purified MBP-μ2 bound to the GluA1–STG complex but not to GluA1 alone ( Fig. 1d , left panels). Similarly, MBP-μ2 bound to the GluA2–STG complex but not to GluA2 alone ( Fig. 1d , right panels). Together, these results indicate that STG facilitates the recruitment of AP-2 to the AMPA receptor complex by directly binding to the μ2 subunit. NMDA induces sequential interaction of STG with AP-2 and -3A To test the possibility that similar to AP-4, AP-2 and AP-3A regulate AMPA receptor trafficking in neurons by binding to STG, we first examined the intracellular localization of STG and AP-2 or AP-3A following NMDA (50 μM) treatment, which induces a ‘chemical LTD’ in hippocampal neurons [7] , [8] , [16] , [17] . At 5 min after the NMDA treatment, Flag-tagged μ2 significantly and maximally co-localized with haemagglutinin (HA)-tagged STG but the co-localization was transient ( Fig. 2a,c ). At 10 min after the NMDA treatment, Flag-μ3A began to co-localize with HA-STG and this interaction continued to increase until at least 20 min after the treatment ( Fig. 2b,c ). These results suggest that STG may change its binding partner from AP-2 to AP-3A during chemical LTD in hippocampal neurons. 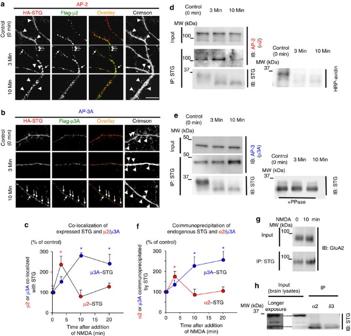Figure 2: Localization of STG and AP-2 or AP-3A following NMDA treatment. (a,b) Immunocytochemical analysis of localization of STG and AP-2 (a) or AP-3A (b) at various time points after NMDA treatment. HA-tagged STG, Flag-tagged μ2 or μ3A and E2-Crimson were coexpressed in hippocampal neurons. Arrows indicate the co-localization of HA-STG and Flag-μ2 (a) or μ3A (b). Arrowheads indicate the spine-like protrusions. Scale bar, 10 μm. (c) Quantitative analysis of STG’s co-localization with μ2 or μ3A;n=5–15 neurons from three independent experiments. *P<0.05 versus time 0 by Student'st-test. Error bars represent means+s.e.m. (d,e) Co-immunoprecipitation assays of the interaction between endogenous STG and endogenous AP-2 (d) or AP-3A (e). At left, lysates of cultured hippocampal neurons were immunoprecipitated using the anti-STG antibody at the indicated time points after NMDA treatment and analysed using antibodies against STG and the α2 subunit of AP-2 (d) or μ3A subunit of AP-3A (e). At the right side ind, the cell surface proteins in hippocampal neurons were biotinylated after NMDA treatment. Lysates were immunoprecipitated using the anti-STG antibody and blotted with horseradish peroxidase (HRP)-conjugated streptavidin. At the right side ine, immunoprecipitated fractions were treated with alkaline phosphatase (PPase) and immunoblotted with the anti-STG antibody. (f) Quantitative analysis of co-immunoprecipitation of endogenous STG with AP-2 or AP-3. The intensities of the bands corresponding to α2 (d) or μ3A (e) that co-immunoprecipitated with STG was normalized to those of immunoprecipitated STG. The ratio of α2/STG or μ3A/STG at time 0 was arbitrarily established as 100% (n=5–11 from three independent experiments). *P<0.05 versus time 0 by Student’st-test. Error bars represent as means+s.e.m. (g) STG does not dissociate from AMPA receptors after NMDA treatment. Hippocampal neurons were treated with NMDA for 10 min and the cell lysates were immunoprecipitated with an anti-GluA2 antibody and immunoblotted with an anti-STG antibody. (h) Endogenous AP-2 or AP-3A binds to the high-mobility form of endogenous STG. Lysates of adult mouse brain were immunoprecipitated with antibodies against α2 or δ3 and analysed using an anti-STG antibody. Figure 2: Localization of STG and AP-2 or AP-3A following NMDA treatment. ( a , b ) Immunocytochemical analysis of localization of STG and AP-2 ( a ) or AP-3A ( b ) at various time points after NMDA treatment. HA-tagged STG, Flag-tagged μ2 or μ3A and E2-Crimson were coexpressed in hippocampal neurons. Arrows indicate the co-localization of HA-STG and Flag-μ2 ( a ) or μ3A ( b ). Arrowheads indicate the spine-like protrusions. Scale bar, 10 μm. ( c ) Quantitative analysis of STG’s co-localization with μ2 or μ3A; n =5–15 neurons from three independent experiments. * P <0.05 versus time 0 by Student's t -test. Error bars represent means+s.e.m. ( d , e ) Co-immunoprecipitation assays of the interaction between endogenous STG and endogenous AP-2 ( d ) or AP-3A ( e ). At left, lysates of cultured hippocampal neurons were immunoprecipitated using the anti-STG antibody at the indicated time points after NMDA treatment and analysed using antibodies against STG and the α2 subunit of AP-2 ( d ) or μ3A subunit of AP-3A ( e ). At the right side in d , the cell surface proteins in hippocampal neurons were biotinylated after NMDA treatment. Lysates were immunoprecipitated using the anti-STG antibody and blotted with horseradish peroxidase (HRP)-conjugated streptavidin. At the right side in e , immunoprecipitated fractions were treated with alkaline phosphatase (PPase) and immunoblotted with the anti-STG antibody. ( f ) Quantitative analysis of co-immunoprecipitation of endogenous STG with AP-2 or AP-3. The intensities of the bands corresponding to α2 ( d ) or μ3A ( e ) that co-immunoprecipitated with STG was normalized to those of immunoprecipitated STG. The ratio of α2/STG or μ3A/STG at time 0 was arbitrarily established as 100% ( n =5–11 from three independent experiments). * P <0.05 versus time 0 by Student’s t -test. Error bars represent as means+s.e.m. ( g ) STG does not dissociate from AMPA receptors after NMDA treatment. Hippocampal neurons were treated with NMDA for 10 min and the cell lysates were immunoprecipitated with an anti-GluA2 antibody and immunoblotted with an anti-STG antibody. ( h ) Endogenous AP-2 or AP-3A binds to the high-mobility form of endogenous STG. Lysates of adult mouse brain were immunoprecipitated with antibodies against α2 or δ3 and analysed using an anti-STG antibody. Full size image To examine whether endogenous STG associates with endogenous AP complexes in a similar time course during LTD, we next performed co-immunoprecipitation assays from cultured hippocampal neurons ( Fig. 2d,e ). The amount of endogenous α-subunits of AP-2 (α2) co-immunoprecipitated with endogenous STG transiently increased at 3 min and returned to control levels at 10 min after NMDA application to hippocampal neurons ( Fig. 2d,f ). In contrast, the amount of endogenous μ-subunits of AP-3A (μ3A) co-immunoprecipitated with STG started to increase at 10 min and remained at high levels at 20 min after NMDA application ( Fig. 2e,f ). These results indicate that endogenous AP–STG interactions occur following NMDA receptor activation in hippocampal neurons ( Fig. 2f ) as observed with overexpression of tagged proteins ( Fig. 2c ). It was previously reported that STG dissociates from the AMPA receptor before endocytosis, when the AMPA receptor is selectively activated by its ligand [18] . Thus, we examined whether the intact STG–AMPA receptor complex was endocytosed after NMDA receptor activation. The cell surface proteins were biotinylated in living neurons 0, 3 and 10 min after NMDA application and cell lysates were immunoprecipitated by an anti-STG antibody. Immunoblot analyses using horseradish peroxidase-conjugated streptavidin revealed that NMDA treatment reduced the amount of STG located at the cell surface ( Fig. 2d , right panels). In addition, immunoblot analysis using an anti-GluA2 antibody revealed that the amount of GluA2 that co-immunoprecipitated with STG was similar before and after NMDA application ( Fig. 2g ). These results indicate that STG does not dissociate from AMPA receptors during NMDA-induced AMPA receptor endocytosis. We observed that STG started to migrate faster on electrophoresis gels at 3 min and the tendency became more apparent at 20 min ( Fig. 2d,e ) after NMDA treatment. To examine whether this phenomenon was caused by the dephosphorylation of STG [12] , STG was immunoprecipitated from neurons after NMDA application and treated with alkaline phosphatase. Immunoblot analysis using an anti-STG antibody revealed that the molecular weight of STG in the control neurons decreased to that of STG in the NMDA-treated neurons ( Fig. 2e , right panels). These results indicate that the higher and lower molecular weight proteins corresponded to the phosphorylated and dephosphorylated forms of STG, respectively. To examine whether endogenous AP-2 and AP-3A also bound specifically to the dephosphorylated form of STG in the brain, we performed co-immunoprecipitation assays from mouse brain lysates using an anti-α2 or anti-δ3 antibody. Immunoblot analyses using an anti-STG antibody showed that the STG that co-immunoprecipitated with AP-2 or AP-3A had a higher mobility than the STG in the input fraction. A longer exposure of the same membrane revealed that a very small amount of STG in the input fraction had a high mobility, similar to that of the STG in the immunoprecipitated fraction ( Fig. 2h ). These results indicate that the high-mobility form of STG, which is likely to correspond to the dephosphorylated form, specifically interacts with AP-2 and AP-3A. Together, these results support the hypothesis that STG mediates the AMPA-receptor trafficking after NMDA receptor activation by STG’s dephosphorylation-dependent recruitment of AP-2 and AP-3A to the AMPA receptor complex. Phosphorylation of STG regulates its binding to AP-2 and -3A To examine whether and how AP–STG interactions are regulated during LTD, we further focused on the STG–CT2 region’s nine conserved serine residues ( Fig. 3a ), which are phosphorylated at basal states and dephosphorylated by the NMDA receptor-mediated activation of calcineurin during hippocampal LTD [12] . We replaced all these serine residues in the CT2 region with alanine (STG 9A ) or aspartate (STG 9D ) to mimic constitutively dephosphorylated or phosphorylated states of STG, respectively, and purified these mutants as GST fusion proteins ( Fig. 3a ). The pull-down assay in HEK293 cells showed that although wild-type STG (STG wt ) and STG 9A bound to both μ2 and μ3A, STG 9D did not bind either one ( Fig. 3b ). The amounts of μ-subunits pulled down by GST 9D were similar to those observed with GST alone or with glutathione beads ( Fig. 3c ). Furthermore, unlike STG wt ( Fig. 1b ), STG 9D did not significantly increase the amount of μ2 subunits that co-immunoprecipitated with GluA1 ( Fig. 3d ). These results indicate that the binding of AP-2 and AP-3A to STG is regulated by STG’s phosphorylation status ( Fig. 3g ). 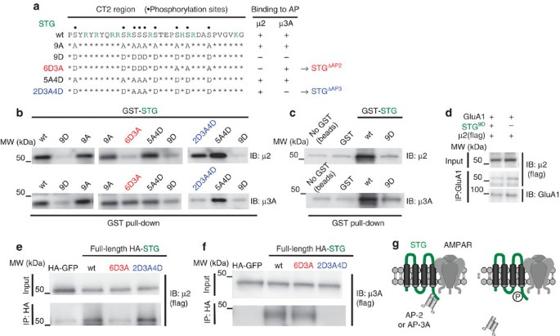Figure 3: Phosphorylation status of STG regulates its binding to AP-2 and AP-3A. (a) Amino acid sequences of the CT2 region of STG and various phospho- and dephosphomimetic STG mutants. Serine residues that can be phosphorylatedin vitroandin vivoare indicated with dots on the top row. Nine basic arginine (R), lysine (K) and histidine (H) residues are shown in bold. Serine was replaced with aspartate or alanine to mimic phosphorylated and dephosphorylated states, respectively. Table at the right side summarizes the results of the GST pull-down assay shown inb. As STG6D3Aand STG2D3A4Dpreferentially lost their binding to μ2 and μ3A, they are designated as STGΔAP2and STGΔAP3, respectively. S, serine; D, aspartate; A, alanine. (b) GST pull-down assay examining the binding of various TARP mutants to μ2 (top) and μ3A (bottom). Lysates of HEK293 cells expressing Flag-tagged μ2 or μ3A were pulled down by the GST-tagged C terminus of wild-type STG (wt) or the indicated STG mutants, and immunoblotted with an anti-Flag antibody. (c) GST pull-down assay examining the background binding of glutathione beads and GST to μ2 (top) or μ3A (bottom). Lysates of HEK293 cells expressing Flag-tagged μ2 or μ3A were pulled down by the GST, glutathione beads alone, GST–STGwtor GST–STG9D, and immunoblotted with an anti-Flag antibody. (d) Co-immunoprecipitation assay of the interaction between GluA1 and μ2 in the presence or absence of phosphomimetic STG. Lysates of HEK293 cells expressing GluA1 and Flag-tagged μ2 were immunoprecipitated using anti-GluA1 and analysed using anti-Flag and anti-GluA1 antibodies. Coexpression of phosphomimetic STG (STG9D) did not enhanced the co-immunoprecipitation of μ2 with GluA1. (e,f) Co-immunoprecipitation assay for the interaction between full-length STG and μ2 (e) or μ3A (f). Lysates of HEK293 cells expressing HA-tagged STG and Flag-tagged μ2 or μ3A were immunoprecipitated using an anti-HA antibody and analysed using an anti-Flag antibody. (g) Schematic drawing of the phosphorylation-dependent interaction of the STG–GluA2 complex with AP-2 or AP-3A. The μ2 or μ3A subunit is incorporated into the STG–GluA2 complex (left), but not when the CT2 region of STG is phosphorylated (right). Figure 3: Phosphorylation status of STG regulates its binding to AP-2 and AP-3A. ( a ) Amino acid sequences of the CT2 region of STG and various phospho- and dephosphomimetic STG mutants. Serine residues that can be phosphorylated in vitro and in vivo are indicated with dots on the top row. Nine basic arginine (R), lysine (K) and histidine (H) residues are shown in bold. Serine was replaced with aspartate or alanine to mimic phosphorylated and dephosphorylated states, respectively. Table at the right side summarizes the results of the GST pull-down assay shown in b . As STG 6D3A and STG 2D3A4D preferentially lost their binding to μ2 and μ3A, they are designated as STG ΔAP2 and STG ΔAP3 , respectively. S, serine; D, aspartate; A, alanine. ( b ) GST pull-down assay examining the binding of various TARP mutants to μ2 (top) and μ3A (bottom). Lysates of HEK293 cells expressing Flag-tagged μ2 or μ3A were pulled down by the GST-tagged C terminus of wild-type STG (wt) or the indicated STG mutants, and immunoblotted with an anti-Flag antibody. ( c ) GST pull-down assay examining the background binding of glutathione beads and GST to μ2 (top) or μ3A (bottom). Lysates of HEK293 cells expressing Flag-tagged μ2 or μ3A were pulled down by the GST, glutathione beads alone, GST–STG wt or GST–STG 9D , and immunoblotted with an anti-Flag antibody. ( d ) Co-immunoprecipitation assay of the interaction between GluA1 and μ2 in the presence or absence of phosphomimetic STG. Lysates of HEK293 cells expressing GluA1 and Flag-tagged μ2 were immunoprecipitated using anti-GluA1 and analysed using anti-Flag and anti-GluA1 antibodies. Coexpression of phosphomimetic STG (STG 9D ) did not enhanced the co-immunoprecipitation of μ2 with GluA1. ( e , f ) Co-immunoprecipitation assay for the interaction between full-length STG and μ2 ( e ) or μ3A ( f ). Lysates of HEK293 cells expressing HA-tagged STG and Flag-tagged μ2 or μ3A were immunoprecipitated using an anti-HA antibody and analysed using an anti-Flag antibody. ( g ) Schematic drawing of the phosphorylation-dependent interaction of the STG–GluA2 complex with AP-2 or AP-3A. The μ2 or μ3A subunit is incorporated into the STG–GluA2 complex (left), but not when the CT2 region of STG is phosphorylated (right). Full size image To assess the difference in the mode of interaction between STG and μ2 or μ3A more precisely, we partially replaced serine residues with alanine or aspartate in the CT2 region of STG, purified them as GST fusion proteins and performed pull-down assays ( Fig. 3a ). Among the various mutants, we found that a mutant STG in which the first six serine residues were replaced with aspartate and the remaining serine with alanine (STG 6D3A ) showed little binding to μ2 but almost normal binding to μ3A ( Fig. 3b ). In contrast, another mutant with serine-to-aspartate substitutions of the first two and last four serine residues and an alanine substitution of the remaining serine (STG 2D3A4D ) showed much weaker binding to μ3A than did STG wt or STG 6D3A , although its binding to μ2 was little affected ( Fig. 3b ). We also performed co-immunoprecipitation assays using full-length wild-type and mutant STG. HA-tagged full-length STG wt was co-immunoprecipitated with Flag-μ2 ( Fig. 3e ) or Flag-μ3A ( Fig. 3f ). In contrast, full-length HA-STG 6D3A was co-immunoprecipitated with Flag-μ3A ( Fig. 3f ) but not with Flag-μ2 ( Fig. 3e ). Conversely, full-length HA-STG 2D3A4D interacted with Flag-μ2 ( Fig. 3e ) but not with Flag-μ3A ( Fig. 3f ). Together, these results indicate that the position of the phosphorylated residues within the CT2 region of STG determines its binding preference for μ2 or μ3A, and that STG uses a different mode of interaction to bind μ2 and μ3A. In the following experiments, we used these STG mutants as tools to examine the role of STG in the AP-2- and AP-3A-mediated trafficking of AMPA receptors in hippocampal neurons. Thus, we designated STG 6D3A and STG 2D3A4D as STG ΔAP2 and STG ΔAP3 , respectively. Binding of STG to AP-2 and -3A is required for AMPAR removal To clarify the role of STG in the regulated transport of AMPA receptors during NMDA-induced chemical LTD, we first coexpressed STG wt , STG ΔAP2 or STG ΔAP3 together with GluA2 to which an HA tag was added to the amino-terminal extracellular domain in cultured hippocampal neurons. After treatment with NMDA (50 μM) for 10 min, the cell surface and total GluA2 were sequentially detected by an anti-HA antibody before and after permeabilizing the plasma membrane. GluA2 immunoreactivity on the cell surface was significantly reduced by the NMDA treatment in neurons expressing STG wt ( Fig. 4a ) and in neurons not expressing any STG constructs ( Supplementary Fig. S2a ). In contrast, the expression of STG ΔAP2 blocked the NMDA-induced reduction of cell surface GluA2 immunoreactivity ( Fig. 4b ). These results indicate that the overexpression of STG ΔAP2 inhibited the NMDA-induced AMPA receptor endocytosis through its dominant-negative effect on the STG–AP-2 interaction. 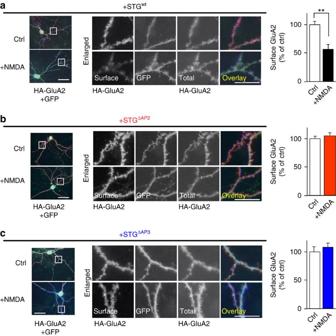Figure 4: Binding of STG to AP-2 and AP-3A is required for the NMDA-induced removal of surface AMPA receptors. (a–c) Immunocytochemical analysis of the effects of wild-type and mutant STG on the NMDA-induced removal of surface AMPA receptors. Cultured hippocampal neurons expressing N-terminal HA-tagged GluA2 and GFP, and STGwt(a), STGΔAP2(b) or STGΔAP3A(c) were treated with 50 μM NMDA for 10 min, fixed and stained for surface HA-GluA2. After permeabilization of the plasma membranes with Triton X, the neurons were stained to detect the total HA-GluA2 level. Regions marked by white squares at the left side are shown at higher magnification at the right side. Scale bars, 20 μm (lower magnification), 10 μm (higher magnification). Graphs at the far right side show the quantitative analysis of the NMDA-induced changes in surface GluA2 immunoreactivity. The ratio of surface HA-GluA2 immunoreactivity was normalized to the total HA-GluA2 immunoreactivity and its value in control neurons (that is, not treated with NMDA) was arbitrarily defined as 100%. **P<0.005 by Student’st-test;n=11–12 cells for each STG construct from three independent experiments. Error bars represent means+s.e.m. Figure 4: Binding of STG to AP-2 and AP-3A is required for the NMDA-induced removal of surface AMPA receptors. ( a – c ) Immunocytochemical analysis of the effects of wild-type and mutant STG on the NMDA-induced removal of surface AMPA receptors. Cultured hippocampal neurons expressing N-terminal HA-tagged GluA2 and GFP, and STG wt ( a ), STG ΔAP2 ( b ) or STG ΔAP3A ( c ) were treated with 50 μM NMDA for 10 min, fixed and stained for surface HA-GluA2. After permeabilization of the plasma membranes with Triton X, the neurons were stained to detect the total HA-GluA2 level. Regions marked by white squares at the left side are shown at higher magnification at the right side. Scale bars, 20 μm (lower magnification), 10 μm (higher magnification). Graphs at the far right side show the quantitative analysis of the NMDA-induced changes in surface GluA2 immunoreactivity. The ratio of surface HA-GluA2 immunoreactivity was normalized to the total HA-GluA2 immunoreactivity and its value in control neurons (that is, not treated with NMDA) was arbitrarily defined as 100%. ** P <0.005 by Student’s t -test; n =11–12 cells for each STG construct from three independent experiments. Error bars represent means+s.e.m. Full size image Interestingly, the expression of STG ΔAP3 , which bound AP-2 but not AP-3A ( Fig. 3b ), blocked the NMDA-induced reduction of cell surface GluA2 immunoreactivity ( Fig. 4c ). The expression of STG ΔAP3 , STG ΔAP2 or STG 9D similarly inhibited the NMDA-induced reduction of surface GluA1 immunoreactivity in hippocampal neurons ( Supplementary Fig. S3 ). In contrast, the AMPA receptor internalization induced by AMPA treatment was not affected by the expression of STG ΔAP2 or STG ΔAP3 ( Supplementary Fig. S4 ), consistent with an earlier report showing that unlike NMDA-induced AMPA receptor endocytosis, the AMPA-induced AMPA receptor endocytosis is independent of AP-2 (ref. 19 ). These results suggest that the NMDA-induced removal of AMPA receptors from the cell surface requires the interaction between STG and AP-3A, as well as the interaction between STG and AP-2. The involvement of AP-2 in AMPA receptor endocytosis has not been directly tested. Thus, to examine the involvement of AP-2, we used the small-interfering RNA (siRNA), which was previously used to knock down the β-subunit of AP-2 (ref. 20 ). Immunoblot analysis of the cell lysates with an anti-HA antibody confirmed that the siRNA directed against AP-2β specifically inhibited expression of co-transfected AP-2β in HEK293 cells ( Supplementary Fig. S5a,b ). Similarly, expression of the siRNA against AP-2β in hippocampal neurons resulted in endogenous AP-2β becoming barely detectable by immunohistochemistry ( Supplementary Fig. S5c ). NMDA treatment did not induce the loss of cell surface GluA2 immunoreactivity in neurons transfected with the siRNA against AP-2β ( Fig. 5a ) but it was induced in neurons transfected with control scrambled siRNA ( Fig. 5b ). To rule out the off-target effect of siRNA, we co-transfected neurons with the siRNA against AP-2β and a complementary DNA encoding a mutant AP-2β resistant to the siRNA, which rescued siRNA-induced reduction of exogenous ( Supplementary Fig. S5a ) and endogenous ( Supplementary Fig. S5e ) AP-2β immunoreactivities. The inhibitory effect of siRNA on NMDA-induced reduction in surface HA-GluA2 immunoreactivity was also rescued by coexpression of the siRNA-resistant AP-2β in hippocampal neurons ( Fig. 5c ). As ablation of one of the four subunits of each AP complex results in total loss of the specific AP complex [14] , [21] , [22] , these results indicate that the AP-2 complex is necessary for NMDA-induced AMPA receptor endocytosis in hippocampal neurons. 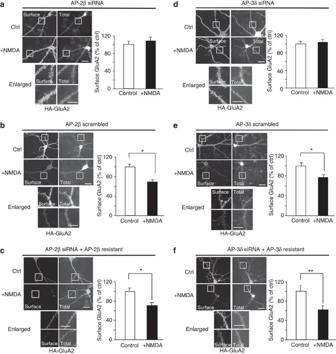Figure 5: Knockdown of AP-2 or AP-3A inhibits the NMDA-induced removal of surface AMPA receptors. (a–c) Immunocytochemical analysis of the effects of knocking down AP-2 on the NMDA-induced reduction of surface GluA2. Cultured hippocampal neurons at 7–10 DIV were transfected with N-terminal HA-tagged GluA2 and siRNA against β2 (a), scrambled control siRNA (b) or siRNA against β2 plus a cDNA encoding an siRNA-resistant β2 (c). At 14–16 DIV, the neurons were treated with NMDA (50 μM) for 10 min, and the surface and total HA-GluA2 were sequentially labelled, that is, before and after membrane permeabilization. The regions marked by white squares are shown at higher magnification at lower panel. Scale bars, 20 μm (lower magnification), 10 μm (higher magnification). (d–f) Immunocytochemical analysis showing the effects of knocking down AP-3A on the NMDA-induced reduction of surface GluA2. Cultured hippocampal neurons were transfected with HA-GluA2 and siRNA against δ (d), scrambled control siRNA (e) or siRNA against δ, plus a cDNA encoding an siRNA-resistant δ (f). After the application of NMDA to the neurons, the surface and total HA-GluA2 were stained. The regions marked by white squares are shown at higher magnification at lower panels. Scale bars, 20 μm (lower magnification), 10 μm (higher magnification). The graphs at the right side show the quantitative analysis of the NMDA-induced changes in surface GluA2 immunoreactivity. *P<0.05 and **P<0.01 by Student’st-test;n=13–16 cells from three independent experiments. Error bars represent means+s.e.m. Figure 5: Knockdown of AP-2 or AP-3A inhibits the NMDA-induced removal of surface AMPA receptors. ( a – c ) Immunocytochemical analysis of the effects of knocking down AP-2 on the NMDA-induced reduction of surface GluA2. Cultured hippocampal neurons at 7–10 DIV were transfected with N-terminal HA-tagged GluA2 and siRNA against β2 ( a ), scrambled control siRNA ( b ) or siRNA against β2 plus a cDNA encoding an siRNA-resistant β2 ( c ). At 14–16 DIV, the neurons were treated with NMDA (50 μM) for 10 min, and the surface and total HA-GluA2 were sequentially labelled, that is, before and after membrane permeabilization. The regions marked by white squares are shown at higher magnification at lower panel. Scale bars, 20 μm (lower magnification), 10 μm (higher magnification). ( d – f ) Immunocytochemical analysis showing the effects of knocking down AP-3A on the NMDA-induced reduction of surface GluA2. Cultured hippocampal neurons were transfected with HA-GluA2 and siRNA against δ ( d ), scrambled control siRNA ( e ) or siRNA against δ, plus a cDNA encoding an siRNA-resistant δ ( f ). After the application of NMDA to the neurons, the surface and total HA-GluA2 were stained. The regions marked by white squares are shown at higher magnification at lower panels. Scale bars, 20 μm (lower magnification), 10 μm (higher magnification). The graphs at the right side show the quantitative analysis of the NMDA-induced changes in surface GluA2 immunoreactivity. * P <0.05 and ** P <0.01 by Student’s t -test; n =13–16 cells from three independent experiments. Error bars represent means+s.e.m. Full size image The function of AP-2β can be partly compensated by a highly similar subunit, AP-1β (ref. 23 ), which is normally incorporated into AP-1. Therefore, to further clarify the specific roles had by AP-2, we knocked down AP-2μ. The NMDA-induced AMPA receptor endocytosis was significantly inhibited in neurons expressing siRNA against AP-2μ but not in those expressing control scrambled siRNA ( Supplementary Fig. S6 ). These data are consistent with those obtained with siRNA against AP-2β ( Fig. 5a–c ). We also examined AP-1’s involvement in the NMDA-induced AMPA receptor endocytosis in hippocampal neurons. GST pull-down assays revealed that AP-1μ bound to the C terminus of STG via the CT2 region ( Supplementary Fig. S7a ). However, the NMDA-induced GluA2 endocytosis appeared normal in the neurons expressing siRNA against AP-1μ ( Supplementary Fig. S7c,d ). These results indicate that AP-2 has a crucial role in the NMDA-induced AMPA receptor endocytosis in hippocampal neurons. Although AMPA receptors are reported to localize at late endosomes/lysosomes after LTD induction [7] , [8] , whether and how AP-3A contributes to NMDA-induced AMPA receptor trafficking remains unclear. Thus, to examine the involvement of AP-3A, we used siRNA against AP-3δ to knock down the δ-subunit of AP-3. Immunoblot analysis of the cell lysates with an anti-HA antibody confirmed that siRNA against AP-3δ specifically inhibited the expression of co-transfected AP-3δ in HEK293 cells ( Supplementary Fig. S5b ). Similarly, the expression of siRNA against AP-3δ inhibited the immunoreactivity of endogenous AP-3δ in hippocampal neurons ( Supplementary Fig. S5d ). NMDA treatment did not induce the loss of cell surface GluA2 immunoreactivity in neurons transfected with the siRNA against AP-3δ ( Fig. 5d ), but this effect was not observed in neurons transfected with control scrambled siRNA ( Fig. 5e ) or in neurons co-transfected with the siRNA and a cDNA encoding a mutant AP-3δ resistant to the siRNA ( Fig. 5f ), indicating that the AP-3A complex is necessary for NMDA-induced removal of cell surface AMPA receptors in hippocampal neurons. Together, these results are consistent with the results obtained using STG ΔAP2 and STG ΔAP3 ( Fig. 4 ), confirming the dominant-negative effects of STG ΔAP2 and STG ΔAP3 on AMPA receptor trafficking. Furthermore, they support the hypothesis that the binding of STG to both AP-2 and AP-3A is required for the NMDA-induced AMPA receptor endocytosis, a chemical LTD model, in hippocampal neurons. AMPAR enters lysosomal pathways by STG–AP-3A interaction As clathrin-dependent endocytosis does not require AP-3A, it was unclear why the NMDA treatment failed to reduce the surface AMPA receptors when the STG–AP-3A interaction was disturbed ( Figs 4c and 5d ). Thus, we performed live imaging to confirm that the AMPA receptor internalization was disrupted in neurons in which AP-2 or AP-3A was knocked down. We expressed GluA2 to which super ecliptic pHluorin (SEP) was attached at the N terminus (SEP-GluA2) and monitored the fluorescence intensity in living hippocampal neurons. As the SEP signal decreases under the low pH conditions in endosomes, a reduction the in SEP signal indicates the endocytosis of surface AMPA receptors. As expected, 10 min after NMDA application, the SEP signal was significantly decreased in control neurons transfected with scrambled siRNA ( Supplementary Fig. S8a,b , left panels). When NH 4 Cl was applied 10 min after NMDA application to neutralize the intracellular acidic compartments, the SEP signal quickly reappeared ( Supplementary Fig. S8a,b , bottom panels), indicating that the SEP-GluA2 was internalized into endosomes. In contrast, NMDA induced little change in the SEP fluorescence in neurons expressing siRNA against AP-2μ ( Supplementary Fig. S8a ) or AP-3δ ( Supplementary Fig. S8b ). These results are consistent with our immunocytochemical analyses ( Fig. 5 ) and indicate that the AMPA receptor internalization observed 10 min after NMDA treatment requires AP-3A. As the number of surface AMPA receptors is determined by the balance between endocytosis and exocytosis (including the recycling of endocytosed receptors), we next used an antibody feeding assay [6] , [10] . HA-GluA2 on the cell surface of living neurons was first labelled with an anti-HA antibody and NMDA was then applied to the neurons to induce HA-GluA2 endocytosis. The anti-HA antibody remaining on the cell surface was then removed by acid treatment; thus, the population of HA-GluA2 that was endocytosed by the NMDA treatment and recycled to the cell surface within 30 min could be specifically visualized; in this assay, HA-GluA2 that does not undergo endocytosis or recycling will not be detected ( Fig. 6a ). There was significantly more recycled GluA2 in neurons expressing STG ΔAP3 than in those expressing STG wt or STG ΔAP2 ( Fig. 6b ). Similarly, immunocytochemical analyses showed that 3 min after NMDA treatment, there was significantly less GluA2 immunoreactivity on the cell surface of neurons expressing STG ΔAP3 or STG wt ( Supplementary Fig. S9a,c ). In contrast, the expression of STG ΔAP2 blocked the NMDA-induced reduction of cell surface GluA2 immunoreactivity even at 3 min ( Supplementary Fig. S9a,c ). These results indicate that AMPA receptors are transiently endocytosed by NMDA treatment but return to the cell surface in neurons expressing STG ΔAP3 , highlighting an important role of the STG–AP-3A interaction in preventing the recycling of endocytosed AMPA receptors. 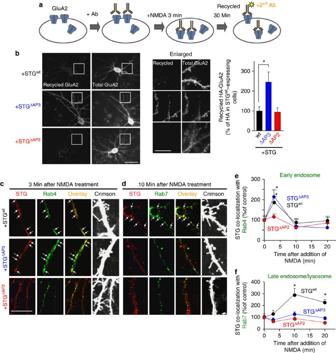Figure 6: Binding of STG to AP-3A is required to prevent recycling of GluA2 to the cell surface. (a) Schematic drawing of the antibody feeding assay. Living neurons expressing N-terminal HA-tagged GluA2 were incubated with an anti-HA antibody and treated with NMDA. After the antibodies remaining on the cell surface were removed by acid treatment, the neurons were incubated for 30 min. GluA2 subunits that were endocytosed and recycled to the cell surface were detected using a secondary antibody. (b) Antibody feeding assay to examine the effects of wild-type and mutant STG on the recycling of GluA2 after NMDA treatment. Cultured hippocampal neurons expressing HA-tagged GluA2 and STGwt, STGΔAP3or STGΔAP2, and subjected to the antibody feeding assay. Scale bar, 20 μm. The regions marked by white squares are shown at higher magnification at the right side. Scale bars, 20 μm (lower magnification), 10 μm (higher magnification). The graphs at the right side show the quantitative analysis of the amount of recycled GluA2 after NMDA treatment. The ratio of recycled HA-GluA2 immunoreactivity was normalized to the total HA-GluA2 immunoreactivity and the ratio in neurons expressing STGwtwas arbitrarily defined as 100%. *P<0.05 by Student’st-test;n=8 cells for each STG construct from two independent experiments. (c,d) Immunocytochemical analysis of STG localization compared with early endosomes (c) and late endosomes/lysosomes (d) after NMDA treatment. Cultured hippocampal neurons were transfected with E2-Crimson, HA-tagged STGwt, STGΔAP3or STGΔAP2, together with GFP-Rab4 (c) or GFP-Rab7 (d). The neurons were treated with NMDA for 0, 3 (c), 10 and 20 min (d), and immunostained for HA and GFP. Arrows indicate the co-localization of HA-STG and GFP-Rab4 (c) or HA-STG and GFP-Rab7 (d). Scale bar, 10 μm. (e,f) Quantitative analysis of STG’s co-localization with Rab4 or Rab7. At 3 min after the NMDA application, STGwtand STGΔAP3, but not STGΔAP2, significantly co-localized with GFP-Rab4 (e). In contrast, only STGwt, but not STGΔAP3or STGΔAP2, started to co-localize with GFP-Rab7 from 10 min after the NMDA application (f). *P<0.05 versus time 0 by one-way ANOVA followed by Tukey’s test;n=6–10 cells. Error bars represent as means+s.e.m. Figure 6: Binding of STG to AP-3A is required to prevent recycling of GluA2 to the cell surface. ( a ) Schematic drawing of the antibody feeding assay. Living neurons expressing N-terminal HA-tagged GluA2 were incubated with an anti-HA antibody and treated with NMDA. After the antibodies remaining on the cell surface were removed by acid treatment, the neurons were incubated for 30 min. GluA2 subunits that were endocytosed and recycled to the cell surface were detected using a secondary antibody. ( b ) Antibody feeding assay to examine the effects of wild-type and mutant STG on the recycling of GluA2 after NMDA treatment. Cultured hippocampal neurons expressing HA-tagged GluA2 and STG wt , STG ΔAP3 or STG ΔAP2 , and subjected to the antibody feeding assay. Scale bar, 20 μm. The regions marked by white squares are shown at higher magnification at the right side. Scale bars, 20 μm (lower magnification), 10 μm (higher magnification). The graphs at the right side show the quantitative analysis of the amount of recycled GluA2 after NMDA treatment. The ratio of recycled HA-GluA2 immunoreactivity was normalized to the total HA-GluA2 immunoreactivity and the ratio in neurons expressing STG wt was arbitrarily defined as 100%. * P <0.05 by Student’s t -test; n =8 cells for each STG construct from two independent experiments. ( c , d ) Immunocytochemical analysis of STG localization compared with early endosomes ( c ) and late endosomes/lysosomes ( d ) after NMDA treatment. Cultured hippocampal neurons were transfected with E2-Crimson, HA-tagged STG wt , STG ΔAP3 or STG ΔAP2 , together with GFP-Rab4 ( c ) or GFP-Rab7 ( d ). The neurons were treated with NMDA for 0, 3 ( c ), 10 and 20 min ( d ), and immunostained for HA and GFP. Arrows indicate the co-localization of HA-STG and GFP-Rab4 ( c ) or HA-STG and GFP-Rab7 ( d ). Scale bar, 10 μm. ( e , f ) Quantitative analysis of STG’s co-localization with Rab4 or Rab7. At 3 min after the NMDA application, STG wt and STG ΔAP3 , but not STG ΔAP2 , significantly co-localized with GFP-Rab4 ( e ). In contrast, only STG wt , but not STG ΔAP3 or STG ΔAP2 , started to co-localize with GFP-Rab7 from 10 min after the NMDA application ( f ). * P <0.05 versus time 0 by one-way ANOVA followed by Tukey’s test; n =6–10 cells. Error bars represent as means+s.e.m. Full size image AP-3A generally mediates the transport of membrane proteins from early endosomes to late endosomes/lysosomes [5] . Thus, STG may regulate AMPA receptor trafficking to this pathway by binding to AP-3A. To test this hypothesis, we examined the location of STG following the NMDA treatment using an early endosome marker, Rab4, tagged with green fluorescent protein (GFP) and a late endosome/lysosome marker, Rab7, tagged with GFP, in hippocampal neurons [24] , [25] . At basal states, the wild-type and mutant STG immunoreactivities rarely co-localized with the GFP-Rab4 ( Supplementary Fig. S10a ) or GFP-Rab7 ( Supplementary Fig. S10b ) signals. However, 3 min after NMDA treatment, STG wt and STG ΔAP3 , but not STG ΔAP2 , co-localized well with GFP-Rab4 ( Fig. 6c,e ), indicating that STG ΔAP2 , which did not interact with AP-2 ( Fig. 3a,b ), was not endocytosed. By 10 min after the NMDA treatment, STG wt , STG ΔAP3 and STG ΔAP2 no longer co-localized with GFP-Rab4 ( Fig. 6c,e ); instead, STG wt started to co-localize with GFP-Rab7 but STG ΔAP3 and STG ΔAP2 did not ( Fig. 6d,f ). Similarly, HA-GluA2 immunoreactivity co-localized with GFP-Rab4 at 3 min after NMDA treatment in neurons expressing STG wt and STG ΔAP3 , but not in neurons expressing STG ΔAP2 ( Supplementary Fig. S11a,c ). From 10 min after the NMDA treatment, HA-GluA2 immunoreactivity started to co-localize with GFP-Rab7 in neurons expressing STG wt , but not in neurons expressing STG ΔAP3 or STG ΔAP2 ( Supplementary Fig. S11b,d ). These results indicate that STG regulates two AMPA receptor transport pathways—transport from the cell surface to the early endosome and from the early endosome to the late endosome/lysosome—by binding to AP-2 and AP-3A, respectively, during NMDA-induced chemical LTD. If the STG–AP-3A interaction mediates AMPA receptor trafficking to the late endosomal/lysosomal pathway during chemical LTD, AMPA receptors that reach the lysosomes might eventually be degraded, although the degradation process could be regulated differently from the trafficking process. To examine this possibility, we analysed whether internalized AMPA receptors were detectable in lysosomes under conditions in which lysosomal proteolysis was inhibited. We coexpressed HA-tagged GluA2 and mCherry-tagged cathepsin B, a lysosomal marker, in cultured hippocampal neurons. After AMPA receptors located at the cell surface were labelled with an anti-HA antibody, the neurons were treated with NMDA for 20 min to induce chemical LTD in the presence of leupeptin, a lysosomal proteolysis inhibitor. Immunocytochemical analyses revealed that the HA-GluA2 became co-localized with the mCherry-cathepsin B signals ( Supplementary Fig. S12a,b ). Importantly, treatment with siRNA against AP-3δ significantly reduced the NMDA-induced co-localization of GluA2 and cathepsin B signals ( Supplementary Fig. S12a,b ). These results indicate that at least a portion of cell surface AMPA receptors on hippocampal neurons are sorted to the lysosomal degradative pathway after LTD induction in an AP-3-dependent manner. We next examined the contribution of the lysosomal degradative pathway to the total GluA2 protein level. The total GluA2 immunoreactivity was similar between hippocampal neurons expressing siRNA against AP-3δ and those expressing a scrambled siRNA ( Supplementary Fig. S12c,d ), indicating that that the basal-state total AMPA receptor level is largely independent of AP-3-dependent degradation pathways. In contrast, NMDA application increased the total GluA2 immunoreactivity level in AP-3δ siRNA-treated hippocampal neurons compared with control neurons ( Supplementary Fig. S12c,d ). These results indicate that the AMPA receptors endocytosed during NMDA-induced LTD are at least partially degraded via AP-3-dependent trafficking to lysosomes. LTD requires the interaction of STG with AP-2 and -3A Finally, to examine the role of STG in the LTD of synaptic transmission, we infected hippocampal CA1 neurons with Sindbis virus encoding GFP and wild-type or mutant STG and performed whole-cell patch–clamp recordings from visually identified CA1 pyramidal neurons in acute slice preparations ( Fig. 7a ). Membrane capacitances of uninfected neurons and neurons expressing STG wt , STG 9D , STG ΔAP2 and STG ΔAP3 were 112±13, 97±9, 108±22, 119±21 and 99±10 pF (mean±s.e.m., n =10 each), respectively. Membrane resistances of uninfected neurons and neurons expressing STG wt , STG 9D , STG ΔAP2 and STG ΔAP3 were 239±18, 213±27, 216±33, 215±18 and 268±34 MΩ ( n =10 each), respectively. These results indicate that expression of wild-type or mutant STG did not affect passive membrane properties of hippocampal neurons. 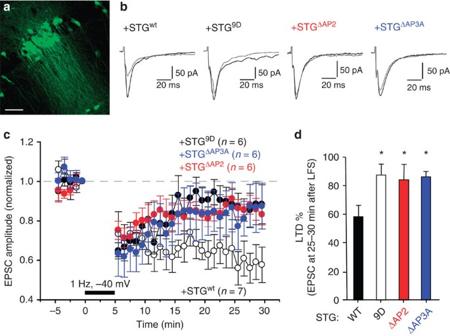Figure 7: Suppression of hippocampal CA1-LTD by inhibiting the interaction of STG with AP-2 or AP-3A. (a) Fluorescence microscopic images of the Sindbis virus-infected hippocampal CA1 pyramidal neurons. Scale bar, 50 μm. (b) Representative SC-evoked EPSCs recorded from CA1 pyramidal neurons expressing STGwt, STG9D, STGΔAP3Aor STGΔAP2just before (solid lines) and 30 min after (grey lines) the application of LFS (1 Hz, 300 stimuli at −40 mV). Holding potential, −80 mV. (c) LTD induction in CA1 pyramidal neurons expressing STGwt, STG9D, STGΔAP3Aor STGΔAP2. EPSC amplitudes were normalized to the amplitudes immediately before LFS and averaged. (d) The diagram showing the averaged EPSC amplitudes at 25–30 min after LFS. STGwt,n=7; STG9D,n=6; STGΔAP2,n=6; STGΔAP3A,n=6. *P<0.05 by the Kruskal–Wallis’s test with the Steel’spost-hoctest. Error bars represent as means±s.e.m. Figure 7: Suppression of hippocampal CA1-LTD by inhibiting the interaction of STG with AP-2 or AP-3A. ( a ) Fluorescence microscopic images of the Sindbis virus-infected hippocampal CA1 pyramidal neurons. Scale bar, 50 μm. ( b ) Representative SC-evoked EPSCs recorded from CA1 pyramidal neurons expressing STG wt , STG 9D , STG ΔAP3A or STG ΔAP2 just before (solid lines) and 30 min after (grey lines) the application of LFS (1 Hz, 300 stimuli at −40 mV). Holding potential, −80 mV. ( c ) LTD induction in CA1 pyramidal neurons expressing STG wt , STG 9D , STG ΔAP3A or STG ΔAP2 . EPSC amplitudes were normalized to the amplitudes immediately before LFS and averaged. ( d ) The diagram showing the averaged EPSC amplitudes at 25–30 min after LFS. STG wt , n =7; STG 9D , n =6; STG ΔAP2 , n =6; STG ΔAP3A , n =6. * P <0.05 by the Kruskal–Wallis’s test with the Steel’s post-hoc test. Error bars represent as means±s.e.m. Full size image Next, we compared the input–output relationship of the Schaffer collateral (SC)-evoked excitatory postsynaptic current (EPSC) amplitudes from CA1 pyramidal neurons in acute slice preparations ( Supplementary Fig. S13a ). We found no difference in the SC–EPSC amplitudes among CA1 neurons expressing wild-type STG, STG ΔAP2 and STG ΔAP3 ( n =7–8 cells each from at least three slices, analysis of variance (ANOVA)). Similarly, no differences were detected in the amplitude or in the rise and decay times of the miniature EPSCs recorded from CA1 neurons expressing wild-type STG, STG ΔAP2 and STG ΔAP3 ( n =7–8 cells each from at least three slices, ANOVA; Supplementary Fig. S13b ). Finally, the AMPA/NMDA ratio, defined as the peak synaptic AMPA receptor current relative to the synaptic NMDA receptor current, was similar among CA1 neurons expressing wild-type STG, STG ΔAP2 and STG ΔAP3 ( n =7–8 cells each from at least three slices, ANOVA; Supplementary Fig. S13c ). Together, these data indicate that the basal synaptic transmission is grossly unaffected by the interaction between STG and AP-2/3. After LFS to the SC (1 Hz, 300 stimuli), LTD was observed in neurons expressing STG wt (the EPSC amplitude at 25–30 min after LFS was 58±8% of baseline, n =7; Fig. 7b–d ) and in uninfected control neurons ( Supplementary Fig. S2b ). In contrast, the LFS-induced LTD was significantly inhibited ( Fig. 7b–d ) in neurons expressing STG 9D (87±8%, n =6, P =0.030 versus STG wt ), STG ΔAP2 (86±4%, n =6, P =0.042 versus STG wt ) or STG ΔAP3A (84±11%, n =6, P =0.030 versus STG wt ; by Kruskal–Wallis’s test with the Steel’s post-hoc test). Although STG ΔAP2 , but not STG ΔAP3A , specifically inhibited trafficking of AMPA receptor–STG complexes to early endosomes at 3 min after NMDA application to cultured hippocampal neurons ( Fig. 6c,e and Supplementary Fig. S6a,c ), we did not observe any difference in EPSC amplitudes (Vh=−40 mV) in neurons expressing STG ΔAP2 and STG ΔAP3A during (23±4% at STG ΔAP2 and 21±4% at STG ΔAP3 , n =6 each, P =0.749 by Mann–Whitney’s U -test) and just after (20±4% at STG ΔAP2 and 17±4% at STG ΔAP3 , n =6 each, P =0.522 by Mann–Whitney’s U -test) LFS. Small differences in EPSC amplitudes could have been masked by transient reduction of EPSC amplitudes observed immediately after LFS application [19] . Nevertheless, these results indicate that the interactions between STG and AP-2, and between STG and AP-3A, are crucial for expression of LFS-induced synaptic LTD in CA1 hippocampal neurons in slices. As the activity-dependent trafficking of AMPA receptors at postsynaptic sites has a central role in experience-dependent plasticity, finding the precise molecular mechanisms that control the trafficking has been a matter of considerable research interest. In this study, we showed that STG mediated the formation of complexes consisting of AMPA receptors and the APs, AP-2 and AP-3A ( Fig. 1 ), in a manner dependent on the dephosphorylation state of STG’s CT2 region ( Fig. 3 ). Both endogenous and overexpressed STG interacted first with AP-2 and then AP-3A during NMDA-induced AMPA receptor endocytosis in hippocampal neurons ( Fig. 2 ). The interaction between STG and AP-2 was required for NMDA-induced AMPA receptor endocytosis, and that between STG and AP-3A was required for the subsequent late endosome/lysosome trafficking of AMPA receptors to prevent them from recycling to the cell surface ( Figs 4 , 5 , 6 ). Similarly, the interactions between STG and AP-2 and AP-3A were necessary for LFS-evoked LTD in CA1 hippocampal neurons ( Fig. 7 ). From these results, we propose a new model in which STG has a critical role in regulating two trafficking pathways of AMPA receptors in hippocampal neurons—transport from the cell surface to early endosomes and from early endosomes to late endosomes/lysosomes—through its sequential binding to AP-2 and AP-3A during NMDA-dependent LTD ( Fig. 8 ). 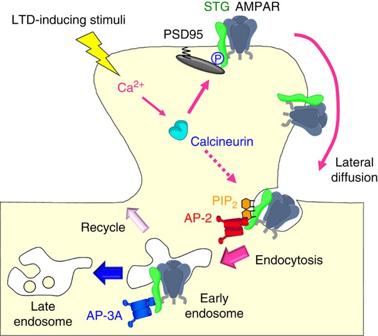Figure 8: A model for the role of STG dephosphorylation in regulating AMPA receptor trafficking during LTD. At postsynaptic sites, PSD-95 binds to STG, which is highly phosphorylated at the C terminus. NMDA receptor-mediated activation of calcineurin during the LTD-inducing stimulus dephosphorylates STG. It is unclear where the dephosphorylation takes place. The AMPA receptor (AMPAR) complex containing dephosphorylated STG may be trapped in the endocytic zone as the complex undergoes lateral diffusion, when the negatively charged lipid PIP2, which is enriched at the endocytic zone, binds to dephosphorylated STG13. Calcineurin also activates production of PIP2at the endocytic zone as shown by the dotted arrow26. As AP-2 also binds PIP2and accumulates at the endocytic zone, the AMPAR complex then enters the clathrin-mediated endocytosis process as a result of the interaction between STG and AP-2. AP-2 is released from endocytic vesicles by the decreased level of PIP2on early endosomes, freeing the C terminus of STG for AP-3A binding, which leads to further trafficking of the complex to late endosomes/lysosomes. When AP-3A cannot bind to STG in early endosomes, the AMPAR complex returns to the cell surface via the recycling pathway. Figure 8: A model for the role of STG dephosphorylation in regulating AMPA receptor trafficking during LTD. At postsynaptic sites, PSD-95 binds to STG, which is highly phosphorylated at the C terminus. NMDA receptor-mediated activation of calcineurin during the LTD-inducing stimulus dephosphorylates STG. It is unclear where the dephosphorylation takes place. The AMPA receptor (AMPAR) complex containing dephosphorylated STG may be trapped in the endocytic zone as the complex undergoes lateral diffusion, when the negatively charged lipid PIP 2 , which is enriched at the endocytic zone, binds to dephosphorylated STG [13] . Calcineurin also activates production of PIP 2 at the endocytic zone as shown by the dotted arrow [26] . As AP-2 also binds PIP 2 and accumulates at the endocytic zone, the AMPAR complex then enters the clathrin-mediated endocytosis process as a result of the interaction between STG and AP-2. AP-2 is released from endocytic vesicles by the decreased level of PIP 2 on early endosomes, freeing the C terminus of STG for AP-3A binding, which leads to further trafficking of the complex to late endosomes/lysosomes. When AP-3A cannot bind to STG in early endosomes, the AMPAR complex returns to the cell surface via the recycling pathway. Full size image The internalization of AMPA receptors is thought to occur through clathrin-mediated endocytosis [10] , [27] , [28] , [29] . Thus, the binding of clathrin adaptor AP-2 to the cargo containing AMPA receptors is a key final step in executing AMPA receptor endocytosis during LTD. Although the μ2 subunit of AP-2 was shown previously to bind directly to the membrane proximal region (MPR) of GluA2/A3 in vitro , in a manner dependent on GluA2’s arginine 845 (R845) [6] , it has been unclear whether and how this process is regulated by neuronal activity. Here we showed that STG bound directly to μ2 and enhanced the formation of a tripartite complex consisting of the AMPA receptor, STG and μ2. As this interaction is dependent on the dephosphorylation of STG that occurs during the NMDA-mediated activation of calcineurin, it nicely explains how AMPA receptors enter the clathrin-mediated endocytosis pathway during LTD. Although an R845A mutation in the MPR of GluA2 disrupts the interaction between the MPR and μ2 (ref. 6 ), our co-immunoprecipitation assay failed to detect differences in the μ2–GluA2 wt and μ2–GluA2 R845A interactions ( Supplementary Fig. S14a ). This is probably because of the different experimental conditions used; Kastning et al. [6] carried out a pull-down assay using a GST-tagged MPR of GluA2 and a recombinant μ2, which was prepared by in vitro transcription and translation, whereas we performed a co-immunoprecipitation assay using full-length GluA2 and μ2 after solubilizing membranes. Thus, a small difference in the μ2–GluA2 wt and μ2–GluA2 R845A interactions may not have been detected in our assay. Nevertheless, STG significantly increased interactions between μ2 and GluA2 by several fold under our experimental conditions ( Fig. 1c ). Interestingly, our co-immunoprecipitation assay indicated that the R845 mutation inhibited the formation of the GluA2–STG–μ2 complex ( Supplementary Fig. S14a ), although both GluA2 wt and GluA2 R845A were similarly co-immunoprecipitated with μ2 ( Supplementary Fig. S14b ). We speculate that the interaction between STG and AP-2 may be regulated allosterically by the binding of the MPR of GluA2 to STG ( Supplementary Fig. S14c ). As endogenous AMPA receptors are tightly associated with STG in vivo , these findings raise the possibility that the inhibitory effects of the R845 mutation of GluA2 on AP-2 binding and on NMDA-induced AMPA receptor endocytosis reported earlier [19] may have been actually mediated indirectly via STG. The atypical μ2-interacting motif within the C2B domain of synaptotagmin contains eight basic amino acids, that is, lysines, arginines and histidines [30] . Interestingly, the CT2 region of STG contains nine basic amino acids and nine serine residues ( Fig. 3a ). Thus, the phosphorylation of the serine residues in the CT2 region probably neutralizes the local charge, thereby inhibiting its interaction with μ2. Furthermore, the MPR of AMPA receptors also contains six basic residues, lysines and arginines. Although the phosphorylation and dephosphorylation of the C terminus of AMPA receptors have essential roles in AMPA receptor trafficking, the mechanism that mediates these effects has remained largely unclear. We postulate that some of the phosphorylation state effects could be mediated by the charge neutralization of the AMPA receptor’s MPR region and/or the TARPs’ CT2 region, to modify the association of AMPA receptor complexes with AP-2 and AP-3A. To understand how AMPA receptor trafficking depends on the phosphorylation status of its GluA subunits, even though TARP binding is not affected by the subunits’ phosphorylation state [31] , further studies are needed to clarify the mechanisms by which the MPR of AMPA receptors and the CT2 region of TARPs interact with each other. Recently, the phosphorylation of STG, which releases STG from the negatively charged lipid bilayers to bind PSD-95, was shown to be necessary for AMPA receptors to enter the postsynaptic site [13] . However, this model does not explain how the dephosphorylation of STG leads to the endocytosis of AMPA receptors during LTD. Although the lipid composition at synapses is currently unclear, phosphoinositide 4,5-bisphosphate (PIP 2 ), a negatively charged lipid, is often enriched at endocytic hot spots [20] , [32] , [33] . Therefore, we propose that the AMPA receptor complex, when released from the postsynaptic site, may be first trapped at the endocytic zone by the STG–PIP 2 interaction ( Fig. 8 ). As the μ2 and α2 subunits of AP-2 also bind PIP 2 and accumulate at the endocytic zone, AMPA receptors may enter the clathrin-mediated endocytic process via the interaction between STG and AP-2 as shown in this study. Interestingly, many APs, including AP-2, also bind simultaneously to both PIP 2 and the cargo protein [32] , [33] . Further studies are necessary to learn how the binding of STG to lipid bilayers and AP-2 is coordinated at synapses. Ten minutes after NMDA treatment, GluA2 co-localizes with Lamp1-positive late endosomes/lysosomes in hippocampal neurons, and lysosomal inhibitors block the NMDA-induced decrease in the total levels of AMPA receptors [7] . Similarly, a very recent paper has reported that expression of a dominant-negative form of Rab7 inhibits LFS-evoked LTD in CA1 hippocampal neurons [34] . Our results on the essential role of late endosomal/lysosomal AMPA receptor trafficking in chemical LTD ( Supplementary Fig. S12 ) and in LFS-evoked LTD in hippocampal slices are consistent with these previous findings. Nevertheless, molecular mechanisms by which the late endosomal/lysosomal trafficking of AMPA receptors during LTD is achieved were unclear. Similarly, although the coexpression of STG 9D prevents GluA1’s entry into the lysosomal degradation pathway [9] , its underlying mechanisms were unknown. Our hypothesis based on the current results successfully provide a molecular explanation for the role of STG in regulating the late endosomal/lysosomal trafficking of AMPA receptors. AP-2 is released from endocytic vesicles by a combination of factors, including a decrease in the level of PIP 2 and dephosphorylation of μ2 on endosomes [35] , [36] . When AP-2 is released, the CT2 region of STG becomes available for AP-3A binding on the early endosome. Alternatively, the partial phosphorylation of STG, as mimicked by STG 6D3A and STG 2D3A4D , may indeed occur in vivo and serve as a molecular rheostat [13] to change its partner from AP-2 to AP-3A. It remains to be determined how the STG–AMPA receptor complex enters the recycling pathway when STG is not able to bind AP-3A. The recycling step may depend on some other adaptor molecule, such as N -ethylmaleimide-sensitive factor, binding to the STG–AMPA complex. Alternatively, recycling to the cell surface might be a default pathway that is activated in the absence of late endosomal/lysosomal trafficking. Our results appear to be at odds with an earlier study arguing that the application of AMPA stimulates the lysosomal degradation of endocytosed AMPA receptors, whereas AMPA receptors internalized by NMDA stimulation rapidly recycle to the cell surface [8] . As previously discussed in detail [7] , this difference could be explained by the use of tetrodotoxin in the earlier study [8] to cause the sustained inhibition of neuronal activity before the application of NMDA; we did not include tetrodotoxin in the present study. Our finding that NMDA promotes the late endosomal/lysosomal trafficking of AMPA receptors is more consistent with the findings that the bath application of NMDA to hippocampal slices causes LTD [17] and that LFS-induced LTD requires NMDA receptor activation [37] , [38] . Nevertheless, the findings of Ehlers [8] indicate that AMPA receptor trafficking could be regulated by other pathways under certain conditions. For example, in mice that lack the genes encoding GluA2 and GluA3 throughout development, the hippocampal LTD is normal, except that it is largely resistant to the dynamin inhibitory peptide [39] , indicating that LTD is no longer mediated by clathrin-dependent endocytosis in these mice. Furthermore, the application of AMPA, but not NMDA, can induce the ubiquitination of AMPA receptors [40] , [41] , [42] , which can be recruited to clathrin-coated pits for endocytosis via the APs epsin and eps15 (ref. 43 ). Therefore, further studies are warranted to clarify whether and how TARPs are involved in the various forms of AMPA receptor trafficking. Chemicals and antibodies NMDA and N -ethyl bromide quaternary salt (QX-314) were purchased from Tocris Bioscience. Picrotoxin was from Sigma. The following antibodies were used: anti-HA antibody (MMS-101P, Covance); anti-FLAG antibody (F7425, Sigma); anti-GluA2 antibody (AB1768), anti-GFP antibody (AB16901) and anti-MAP2 antibody (AB5622, Chemicon); anti-GluA1 antibody (06-306, Upstate); and anti-STG antibody (C8206, Sigma). Construction and transfection or transformation of plasmids Utilizing PCR with Pyrobest DNA polymerase (Takara, Tokyo, Japan), cDNA encoding an HA, Flag or GFP was added to the 5′-end (immediately following the signal sequence) or 3′-end (immediately upstream of the stop codon) of mouse GluA1, full-length TARP, μ2 or μ3A cDNA. Similarly, cDNAs encoding a far-red fluorescent protein E2-Crimson (Clontech) followed by a self-cleaving 2A peptide from foot-and-mouse-disease virus [44] were added to the 5′-end of full-length TARP. The nucleotide sequences of the amplified open reading frames were confirmed by bidirectional sequencing. After the cDNAs were cloned into expression vectors, either pTracer (Invitrogen) or pCAGGS (provided by Dr J Miyazaki, Osaka University, Osaka, Japan), the constructs were transfected into HEK293 cells using the CellPhect transfection kit (Amersham Pharmacia) or into hippocampal neurons using Lipofectamine 2000 (Invitrogen) following the manufacturers’ instructions. For the expression of GST fusion proteins, the cDNA encoding the C terminal region of each wild-type or mutant TARP was amplified by PCR and cloned into pGEX 4T-2. Escherichia coli BL21 (DE3) were transformed with these pGEX expression vectors and the expression of GST fusion proteins was induced by the addition of 0.1 mM isopropyl-β- D -thiogalactoside. Culture of hippocampal neurons Hippocampi dissected from E16-E17 ICR mice were treated with 10 U ml −1 trypsin and 100 U ml −1 DNase in DMEM medium (Sigma) at 37 °C for 20 min. The dissociated hippocampal neurons were plated on polyethyleneimine-coated plates or glass coverslips and cultured in neurobasal medium (Invitrogen) with NS21 supplement [45] and 0.5 mM L-glutamine. After 7–10 days in vitro (DIV), the neurons were transiently transfected with plasmids using Lipofectamine 2000 following manufacturer’s instructions. Briefly, 2 μg of plasmid DNA was mixed with 2 μl of Lipofectamine 2000 in 200 μl of DMEM. After 20-min incubation at room temperature, the mixtures were added to hippocampal neurons. All procedures relating to the care and treatment of animals were performed in accordance with NIH guidelines and permitted by Keio University Experimental Animal Committee. Co-localization assay For detecting co-localization of STG and AP-2 or AP-3, hippocampal neurons were transfected with HA-tagged STG, Flag-tagged μ2 or μ3A, and a far-red fluorescent protein E2-Crimson to distinguish structural details of neurons. For detecting co-localization of STG and Rab, GFP-tagged Rab4 or Rab7 was used instead of μ2 or μ3A. Neurons were stimulated with 50 μM NMDA for 10 min, fixed in 4% paraformaldehyde for 10 min at room temperature, immunostained with the anti-HA antibody (1:1,000) and anti-Flag or anti-GFP antibody (1:1,000), which were visualized with Alexa 546 and Alexa 488 secondary antibodies (1:1,000), respectively. For detecting co-localization of internalized GluA2 and cathepsin, HA-tagged GluA2 and mCherry-tagged cathepsin were expressed in cultured hippocampal neurons. Cell surface HA-GluA2 was labelled with an anti-HA antibody (1:100) for 1 h in living hippocampal neurons. The neurons were then treated with 50 μM NMDA for 20 min and fixed in 4% paraformaldehyde for 10 min at room temperature. HA-GluA2 labelled with an anti-HA antibody was visualized by an Alexa 488-conjugated secondary antibody (1:1,000). Fluorescence images were captured by confocal microscopy (FV1000, Olympus) under the same settings. We selected well-branched spiny mature neurons and analysed using IP-lab software (Scanalytics). A macro script utilizing an autosegmentation filter was used to define segments. STG- or cathepsin-immunopositive regions were defined as segments whose red fluorescence intensities were >50. The co-localized regions were defined as segments whose yellow fluorescent intensities were >50. The co-localization ratio was then calculated by dividing total area of co-localized (yellow) segments by that of STG or cathepsin (red) segments. The averaged co-localization ratio calculated from control neurons without NMDA treatment in sister cultures was arbitrarily established as 100%. Assay for AMPA receptor endocytosis Hippocampal neurons transfected with plasmids for HA-GluA2 and wild-type or mutant STGs were stimulated with 50 μM NMDA for 10 min and fixed in 4% paraformaldehyde without permeabilization for 10 min at room temperature. After the fixed neurons were washed with PBS and incubated with a blocking solution (2% BSA and 2% normal goat serum in PBS), the surface HA-GluA2 was labelled with the anti-HA antibody (1:1,000) and an Alexa 546-secondary antibody (1:1,000). To examine whether the plasma membrane of neurons was intact, neurons were labelled with an antibody against MAP2, an intracellular protein, under non-permeabilizing conditions, and then with the Alexa 488-secondary antibody (1:1,000). To label the total HA-GluA2, the neurons were then permeabilized and blocked with the blocking solution containing 0.4% Triton X-100 and were incubated with the anti-HA antibody (1:1,000) and an Alexa 350 secondary antibody (1:1,000). GFP protein expression was also detected by anti-GFP (1:3,000) and Alexa 488 (1:1,000) antibodies. Fluorescence images were captured by a fluorescence microscope (BX60, Olympus) equipped with a charge-coupled device camera (DP 70, Olympus) and analysed using IP-Lab software. For the statistical analysis of the surface expression level of HA-GluA2, only transfected neurons with well-differentiated dendrites and spines were chosen. Neurons that showed MAP2 immunoreactivity under non-permeabilizing conditions were excluded from quantitative assays. As the amount of protein in the somatic region was sometimes very high, the immunoreactivities were measured between 20 and 100 μm from the soma. The intensity of the immunoreactivity for surface HA (Alexa 546) in the dendrites of the hippocampal neurons was normalized using the value of the intracellular HA immunoreactivity (Alexa 350). The averaged surface/total ratio calculated from control neurons without NMDA treatment in sister cultures was arbitrarily established as 100%. For the cell surface biotinylation assay of STG, hippocampal neurons at 17 DIV were treated with NMDA for 0, 3 or 10 min at room temperature and the cell surface proteins were biotinylated using EZ-Link Sulfo-NHS-Biotinylation Kit (Thermo Fisher Scientific) at 4 °C for 30 min. Next, cell lysates were immunoprecipitated with an anti-GluA2 antibody and immunoblotted with an anti-STG antibody. For live imaging of AMPA receptor endocytosis, we expressed GluA2 to which super ecliptic pHluorin was attached at the N terminus (SEP-GluA2), together with scrambled RNA or siRNA against the μ-subunit of AP-2 or the δ-subunit of AP-3A. After 50 μM NMDA was applied to living neurons for 10 min, the SEP fluorescence was analysed by confocal microscopy (D-ECLIPSE C-1, Nikon). NH 4 Cl (5 mM) was then applied to neurons to detect the SEP-GluA2 in intracellular acidic compartments. Assay for AMPA receptor recycling Living hippocampal neurons transfected with plasmids for HA-GluA2 and wild-type or mutant TARPs were labelled with the anti-HA antibody (1:100) for 1 h. After washing out excess antibodies, the neurons were stimulated with 50 μM NMDA for 3 min. The NMDA was washed out and the neurons were incubated for 30 min at 37 °C, fixed in 4% paraformaldehyde without permeabilization for 10 min at room temperature, washed with PBS and incubated with a blocking solution (2% BSA and 2% normal goat serum in PBS). The surface HA antibody was visualized with an Alexa 546-secondary antibody (1:1,000). To label the total HA-GluA2, the neurons were then permeabilized and blocked with blocking solution containing 0.4% Triton X-100 and then incubated with the anti-HA antibody (1:1,000) and Alexa 350 secondary antibody (1:1,000). Fluorescence images were captured by a fluorescence microscope equipped with a charge-coupled device camera and analysed using IP-Lab software. For statistical analysis of the recycled HA-GluA2, the intensity of Alexa 546 for recycled HA-GluA2 was measured and normalized to the intensity of Alexa 350 for total HA-tagged GluA2. The fluorescence intensity on dendrites between 20 μm and 100 μm from the soma was measured. Pull-down and co-immunoprecipitation assays The C terminus of wild-type and mutant STGs were purified as GST fusion proteins (GST–STG) and added to the lysates of HEK293 cells expressing the μ-subunits of APs. In some experiments, GST–STG was mixed with the purified μ2 subunit of AP-2, which was prepared as a fusion protein with MBP-μ2. After a 1 h incubation at 4 °C, GST proteins were pulled down by glutathione sepharose resin (Amersham Pharmacia) and the precipitates were analysed by immunoblotting. For co-immunoprecipitation assays, transfected HEK293 cells were solubilized in 500 μl of TNE buffer (50 mM NaCl, 10% NP-40, 20 mM EDTA, 0.1% SDS, 50 mM Tris-HCl, pH 8.0) supplemented with a protease inhibitor cocktail (Calbiochem). For co-immunoprecipitation, 1.2 μg of anti-GluA1 antibody, 1.2 μg of anti-GluA2 antibody or 3.0 μg of anti-STG antibody was added to the cell lysates and the mixture was incubated for 1 h at 4 °C. Next, 50 μl of protein G-conjugated agarose (Amersham Pharmacia) was added and this mixture was incubated for 1 h at 4 °C. The precipitates were washed four times with 500 μl of TNE buffer, then 50 μl of SDS–PAGE sample buffer was added and the samples were incubated for 5 min at 95 °C. After centrifugation, 5 μl of the supernatant was analysed by immunoblotting with anti-Flag (Sigma) or other primary antibodies, followed by a TrueBlot horseradish peroxidase-conjugated secondary antibody (eBioscience) and the ECL plus reagents (Amersham Pharmacia). To reduce variations caused by subtle differences in experimental conditions, such as cell properties and transfection efficiency, we performed co-immunoprecipitation assays using just two samples at the same time, one for test and one for control, from sister cultured cells [14] . For example, cells in one dish were transfected with test cDNAs consisting of GluA1, μ2 and STG, and sister cultured cells in another dish were transfected with control cDNAs consisting of GluA1 and μ2 without STG. Co-immunoprecipitation and immunoblot analyses were performed on this paired samples at the same time. The band intensities were quantified using an image analyser (LAS-3000 mini, Fuji Photofilm). The co-immunoprecipitation ratio was calculated by dividing the intensity of the band in the co-immunoprecipitated fraction by the intensity of the respective molecule in the input lysate. The co-immunoprecipitation ratio of the test sample was then normalized to that of the control sample in the same set of experiment. After repeating such independent pairwise experiments, the normalized co-immunoprecipitation ratios were combined. Full-sized scans of key western blottings are provided in Supplementary Fig. S15 . Knockdown of AP-2 and AP-3A The nucleotide sequence for the siRNA against mouse AP-1μ [46] , AP-2μ [47] and AP-2β [20] was previously reported. The siRNA for mouse AP-3δ was generated by Sigma Genosys. The corresponding 19-nt sequence was as follows: 5′-GUG AGA AGC UGC CUG UCC A-3′. For rescue experiments, five nucleotides (AP-2β) and seven nucleotides (AP-3δ) were mutated in the region targeted by siRNAs without changing the amino acid sequence to generate mutant AP-2β and AP-3δ resistant to siRNAs. Hippocampal neurons were transfected with siRNA and plasmids at 10 DIV using Transmessenger (Qiagen) according to the manufacturer’s instruction. The transfection mixture consisted of 0.1 μg siRNA, 0.2 μg plasmid DNA, 2.4 μl Enhancer R and 1.5 μl Transmessenger reagent in 100 μl of neurobasal medium (Invitrogen) with NS21 supplement. Recombinant Sindbis virus and in vivo injection The recombinant Sindbis virus used for the expression of STG in combination with GFP was constructed as described [14] . Under deep anaesthesia with an intraperitoneal injection of ketamine/xylazine (80/20 mg kg −1 , Sigma), the solution containing the recombinant Sindbis virus (2.5 μl; titre, 1.0 × 10 8−9 TU ml −1 ) was injected into the CA1 region of the dorsal hippocampus of ICR mice aged postnatal day 14–22 stereotaxically (2.0–2.3 mm posterior to the Bregma, 1.5−2.0 mm lateral to the midline and 1.5–2.0 mm ventral from the pial surface). Twenty-four hours after injection, the infected cells were identified by their GFP expression. Electrophysiology Transverse hippocampal slices (250-μm thickness) were prepared from the infected ICR mice 24 h after Sindbis virus injection and whole-cell patch–clamp recordings were made from CA1 pyramidal cells that emitted GFP fluorescence, using an Axopatch 200B amplifier (Molecular Devices) and the pCLAMP system (version 9.2, Molecular Devices) at room temperature. The resistance of patch pipettes was 4–6 MΩ when the samples were filled with an intracellular solution consisting of 150 mM Cs-gluconate, 10 mM HEPES–NaOH (pH 7.3), 8 mM MgCl 2 , 2 mM Na 2 ATP, 0.5 mM Na 2 GTP, 0.2 mM EGTA and 5 mM QX-314 (290 mOsm kg −1 ). The solution used for slice storage and recording consisted of 125 mM NaCl, 2.5 mM KCl, 2 mM CaCl 2 , 1 mM MgCl 2 , 1.25 mM NaH 2 PO 4 , 26 mM NaHCO 3 and 10 mM D -glucose, which was bubbled continuously with a mixture of 95% O 2 and 5% CO 2 . Picrotoxin (100 μM) was always added to the assay to block inhibitory synaptic transmission. To evoke EPSCs, SCs were stimulated by a glass stimulating electrode placed on the stratum radiatum of the CA1 region. For LTD experiments, EPSCs were recorded successively at a frequency of 0.1 Hz from CA1 pyramidal neurons voltage-clamped at −80 mV. After stable EPSCs were observed for at least 5 min, the LFS (1 Hz, 300 stimuli at −40 mV) was applied. Access resistances were monitored every 10 s by measuring the peak currents in response to 2-mV, 50-ms hyperpolarizing steps throughout the experiments; the measurements were discarded if the resistance changed by >20% of its original value. Current responses were filtered at 1 kHz and digitized at 4 kHz. Statistical analysis Data were analysed using two-sided Student’s t -test, the Mann–Whitney’s U -test, the Kruskal–Wallis’s test with the Steel’s post-hoc test and one-way ANOVA with the Tukey’s honestly significant difference post-hoc test. How to cite this article: Matsuda, S. et al. Stargazin regulates AMPA receptor trafficking through adaptor protein complexes during long-term depression. Nat. Commun. 4:2759 doi: 10.1038/ncomms3759 (2013).